Formation of titanium monoxide (001) single-crystalline thin film induced by ion bombardment of titanium dioxide (110) A plethora of technological applications justify why titanium dioxide is probably the most studied oxide, and an optimal exploitation of its properties quite frequently requires a controlled modification of the surface. Low-energy ion bombardment is one of the most extended techniques for this purpose and has been recently used in titanium oxides, among other applications, to favour resistive switching mechanisms or to form transparent conductive layers. Surfaces modified in this way are frequently described as reduced and defective, with a high density of oxygen vacancies. Here we show, at variance with this view, that high ion doses on rutile titanium dioxide (110) induce its transformation into a nanometric and single-crystalline titanium monoxide (001) thin film with rocksalt structure. The discovery of this ability may pave the way to new technical applications of ion bombardment not previously reported, which can be used to fabricate heterostructures and interfaces. Low-energy ion bombardment (LEIB) is a common tool to achieve the controlled generation of surface defects and self-organized nanostructures [1] , [2] , [3] . In this sense, oxides are interesting targets for ion-induced modifications, as their tolerance to non-stoichiometry allows the exploration of a wide range of induced morphologies and properties. In particular, TiO 2 , which is a model system in many investigations [4] , is also the subject of a large number of studies in this direction, where the formation of nanoripples [5] or rough surfaces [6] has been reported after irradiation with high ion doses. Besides resistive switching [7] , [8] , ion bombardment has been also recently utilized to achieve a proper response of the optical and electric [9] , [10] properties of surfaces with the aim of improving light emission [11] or magnetotransport [12] , [13] . In these cases titanium suboxides play a pre-eminent role. To name a few examples, recent works have proposed a memristor specifically based on TiO (ref. 14 ), a heavily bombarded TiO 2 (110) surface [8] as an optimal substrate for resistive switching writing at the nanoscale, and a bombarded TiO 2 (100) surface [10] as a nanometric transparent semiconductor. But, despite the intensive use of LEIB in oxides, a detailed study of the modified structure at the atomic level on ion bombardment is, surprisingly, still lacking. This situation is undesirable, as all physical properties depend ultimately on the structure. We show in this context that, under the proper conditions, the surface of an ion-bombarded oxide is not necessarily converted into the defective or amorphous version of the oxide, but can be rather transformed into a single-crystalline thin film of the corresponding suboxide. Experimental results The as-prepared flat TiO 2 samples show, before ion erosion, atomically flat terraces separated by monoatomic steps. After the bombardment (carried out with Ar + , with an ion energy of E =3 keV, under normal incidence and at room temperature), the surfaces show a rough topography with no recognizable pattern or symmetry. No ripples or similar types of nanostructures form under the experimental conditions employed (see Supplementary Fig. 1 ). However, X-ray diffraction (XRD), in conventional θ −2 θ scans, shows the emergence of a new single reflection, consistent with TiO(002), which is not present in the pristine surface ( Fig. 1a ). The (001) interplanar separation measured is d z =2.08 Å. Thus, the formation of crystalline TiO, which is not randomly oriented, but with its [001] direction aligned along the [110] direction of TiO 2 , is clearly induced by ion bombardment. For lower ion doses, the intensity of the (002) reflection of TiO is, as expected, much smaller, whereas the interplanar distance is reduced to d z =2.04 Å. 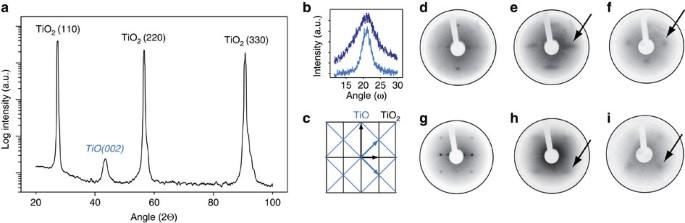Figure 1: X-ray diffraction and low-energy electron diffraction studies. (a)θ–2θScan taken after ion bombardment, where a new reflection assigned to TiO(002) is present. (b) Rocking scans of the TiO(002) reflection around the [001] (dark blue) and [10] (light blue) axis of TiO2. (c) Scheme of the surface unit cells and lattices in reciprocal space for TiO (blue) and TiO2(black), as deduced from the LEED patterns. (d–f) Series of consecutive LEED patterns (taken at an electron energy of 63 eV) of the TiO2(110) surface before ion bombardment (d), after ion bombardment (e) and after a mild annealing of the bombarded surface (f). (g–i) The same as the previous (d–f) LEED patterns, but taken at an electron energy of 95 eV. The arrows are guides that point to the diffuse main reflections of the TiO(001) surface. Figure 1: X-ray diffraction and low-energy electron diffraction studies. ( a ) θ –2 θ Scan taken after ion bombardment, where a new reflection assigned to TiO(002) is present. ( b ) Rocking scans of the TiO(002) reflection around the [001] (dark blue) and [10] (light blue) axis of TiO 2 . ( c ) Scheme of the surface unit cells and lattices in reciprocal space for TiO (blue) and TiO 2 (black), as deduced from the LEED patterns. ( d – f ) Series of consecutive LEED patterns (taken at an electron energy of 63 eV) of the TiO 2 (110) surface before ion bombardment ( d ), after ion bombardment ( e ) and after a mild annealing of the bombarded surface ( f ). ( g – i ) The same as the previous ( d – f ) LEED patterns, but taken at an electron energy of 95 eV. The arrows are guides that point to the diffuse main reflections of the TiO(001) surface. Full size image To check the crystallinity of the induced phase in long lateral length scales, we have measured rocking curves around the TiO(002) reflection along the two main axis of the TiO 2 (110) single crystal: the [10] and [001] high symmetry directions. The results show ( Fig. 1b ) broad rocking curves with different FWHM: Δω 1−10 =3.0° and Δω 001 =6.8°. These values can be compared with the typical FWHM ( Δ ω TiO 2 ≈ 0.04°) of a rocking curve in the TiO 2 single crystal. Thus, a relatively high tilting of the TiO crystal with respect to the TiO 2 (110) crystal is present around both in-plane axis, albeit it is higher around the [001] direction than around the [10] axis (the directions are always those of the TiO 2 (110) crystal). Low-energy electron diffraction (LEED) experiments have been performed during ion bombardment and immediately after it. The pristine surface shows the typical pattern of the (1 × 1)-TiO 2 (110) structure, with sharp spots and a dark background ( Fig. 1d,g ). In the early stages of ion bombardment, the LEED pattern completely disappears, giving rise to a diffuse background with no discernable spots. At higher doses, new spots emerge, which are very broad, diffuse and elongated along the [10] direction of the TiO 2 surface ( Fig. 1e,h ). This is in agreement with the asymmetry observed in the X-ray rocking curves. A thermal annealing of the sample up to around 100 °C transforms the elongated spots into more symmetrical and better-defined reflections ( Fig. 1f,i ), thus suggesting an improvement of the crystalline order of the topmost layers of the induced TiO phase. Figure 1c shows the reciprocal unit cell, as indicated by the LEED patterns. The new lattice reflects a square unit cell (as projected onto the surface) rotated 45° with respect to the surface unit cell of the rutile. The surface lattice parameters are fully compatible (within the uncertainty due to the broadness of the diffraction spots) with the 4.18 Å of the tabulated lattice parameter of TiO. Thus, the developed LEED pattern also confirms the existence of a TiO(001) phase, which is in registry with the rutile lattice. Interestingly, this phase emerges after long ion doses and after a transient state where the surface is disordered as no diffraction pattern is perceived. This behaviour is opposed to the case of metals for which, under similar ion fluencies, intensively bombarded surfaces always show a clear LEED pattern [15] , [16] . From the chemical point of view, the most evident effect produced by ion bombardment is the reduction of Ti in the region close to the surface, which is a well-known phenomenon in oxides. Preferential sputtering of a given element frequently occurs in multicomponent materials, mainly due to the different masses (different efficiencies for energy transfer during collisions) and bonding energies of the elements [17] . In oxides, oxygen atoms are usually preferentially ejected. In particular, numerous experimental works in TiO 2 have provided clear evidences of the chemical reduction of the surfaces [6] , [18] , [19] , [20] , [21] . In all the cases studied, TiO 2 looses oxygen during LEIB. This is confirmed in our case by Auger spectra displaying a shoulder at higher electron energies in the LMV and MNN peaks, signifying a high concentration of Ti 2+ species ( Supplementary Fig. 2 ). The nominal stoichiometry of the surface is found to be TiO 1.2 . Therefore, under the current experimental conditions, the reduction towards TiO is not complete and, besides the most abundant Ti 2+ , there is a number of Ti 3+ and Ti 4+ cations in the vicinity of the surface. We have used atomic resolution scanning transmission electron microscopy (STEM) to analyse the local structure of the films. Low-magnification high-angle annular dark field and annular bright field images of samples oriented with the electron beam parallel to the [001] axis ( Fig. 2a,b ) show a flat irradiated layer. Its thickness is ~10 nm, being very homogeneous over long lateral length scales. High-magnification images for the same orientation ( Fig. 2c,d ) confirm the flatness of the interface between the substrate and the irradiated layer (not atomically sharp, though). The irradiated layer exhibits a high degree of crystalline order with short range order within a few nanometres, and a well-defined orientation relative to the underlying substrate (see insets in Fig. 2c , both in real and in Fourier spaces). These findings are fully consistent with the structural analysis previously explained (see also Supplementary Notes and Supplementary Fig. 4 ). 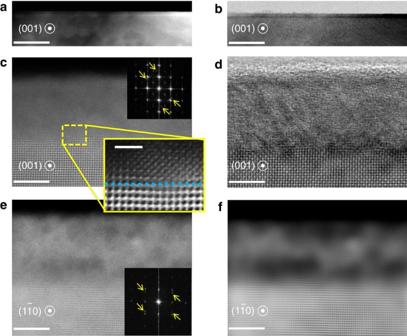Figure 2: Electron microscopy characterization of the irradiated film. (a,b) High-angle annular dark field (HADF) (Z-contrast) (a) and annular bright field (ABF) (b) low-magnification images of the irradiated layer along the [001] direction. (c,d) High-magnification HADF (c) and ABF (d) images for the same orientation. The lower inset incshows more clearly the partially coherent interfaces between the TiO2substrate and the irradiated layer. A horizontal dotted blue line marks the interface position. The white scale length is 2 nm. The upper inset in (c) shows the Fast Fourier Transform (FFT) extracted from the whole image, where the spots at the yellow arrows correspond to the TiO layer. They show a tilting of the lattice of a few degrees for the specific area scanned, in agreement with the tilting observed with diffraction techniques along the [001] direction of TiO2(Fig. 1). (e) High-magnification HADF image along the [10] orientation. The inset in (e) shows the FFT extracted from the whole image. Yellow arrows point at the reflections of the TiO thin film. (f) HADF filtered image from (e). The white scale bars are 100 nm for (a,b) and 5 nm for (c–f). Figure 2: Electron microscopy characterization of the irradiated film. ( a , b ) High-angle annular dark field (HADF) ( Z -contrast) ( a ) and annular bright field (ABF) ( b ) low-magnification images of the irradiated layer along the [001] direction. ( c , d ) High-magnification HADF ( c ) and ABF ( d ) images for the same orientation. The lower inset in c shows more clearly the partially coherent interfaces between the TiO 2 substrate and the irradiated layer. A horizontal dotted blue line marks the interface position. The white scale length is 2 nm. The upper inset in ( c ) shows the Fast Fourier Transform (FFT) extracted from the whole image, where the spots at the yellow arrows correspond to the TiO layer. They show a tilting of the lattice of a few degrees for the specific area scanned, in agreement with the tilting observed with diffraction techniques along the [001] direction of TiO 2 ( Fig. 1 ). ( e ) High-magnification HADF image along the [10] orientation. The inset in ( e ) shows the FFT extracted from the whole image. Yellow arrows point at the reflections of the TiO thin film. ( f ) HADF filtered image from ( e ). The white scale bars are 100 nm for ( a , b ) and 5 nm for ( c – f ). Full size image A more complete view of the induced structure can be achieved with Grazing Incidence XRD (GIXRD) measurements. The pristine surface just shows the reflections of the rutile unit cell, but new reflections are clearly present in the modified surface. 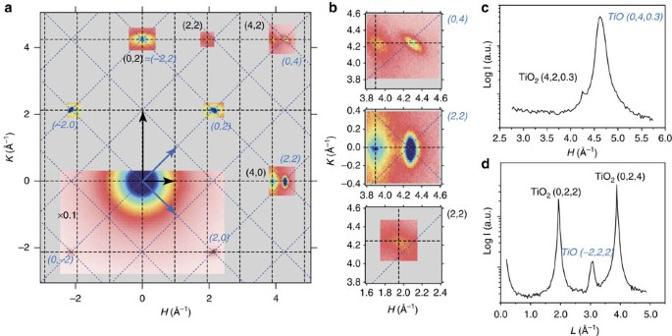Figure 3: Surface X-ray diffraction studies of the modified TiO2(110) surface. (a) HK map in reciprocal space, taken atL=0.3 Å−1, where both sets of reflections for the two observed structures, TiO2and TiO, are present. The TiO2lattice and indexed reflections are coloured in black, while those of the rocksalt TiO lattice are shown in blue italic for all the figures. The large dark blue area at (H,K)=(0,0) is not a real Bragg reflection but part of the direct beam. The displayed intensity in the large matrix below has been divided by a factor of 10. (b) Details of some reflections appearing in (a) corresponding to both the TiO2and TiO crystals. (c,d)H- andL-scans of the modified surface. In both cases new reflections corresponding to the TiO lattice emerge, which were not initially present in the pristine surfaces. These reflections determine the in-plane (c) and out-of-plane (d) periodicities of the new crystalline structure. Figure 3a shows a HK scan in reciprocal space. The scan shows (0,2), (0,4) and (2,2) reflections of a square lattice, which all accurately correspond to the relaxed rocksalt TiO(001) orientation rotated 45° with respect to the rutile surface unit cell, as already observed by LEED. Other reflections are those of the rutile (110) cell not subjected to extinction rules. Some are obscured by the much broader reflections of the TiO lattice. To get the out-of-plane periodicity of the induced rocksalt structure, we have carried out L -scans ( Fig. 3d ), which show a new reflection at L =3.04 Å −1 that nicely agrees with 2 π / d z . It is worth remarking that before and during GIXRD experiments the sample was exposed to air for several days, which denotes the robustness of the thin film under ambient conditions. Figure 3: Surface X-ray diffraction studies of the modified TiO 2 (110) surface. ( a ) HK map in reciprocal space, taken at L =0.3 Å −1 , where both sets of reflections for the two observed structures, TiO 2 and TiO, are present. The TiO 2 lattice and indexed reflections are coloured in black, while those of the rocksalt TiO lattice are shown in blue italic for all the figures. The large dark blue area at (H,K)=(0,0) is not a real Bragg reflection but part of the direct beam. The displayed intensity in the large matrix below has been divided by a factor of 10. ( b ) Details of some reflections appearing in ( a ) corresponding to both the TiO 2 and TiO crystals. ( c , d ) H - and L -scans of the modified surface. In both cases new reflections corresponding to the TiO lattice emerge, which were not initially present in the pristine surfaces. These reflections determine the in-plane ( c ) and out-of-plane ( d ) periodicities of the new crystalline structure. Full size image Density functional theory calculations To assess the atomic structure and stability of the interface between the TiO(001) and TiO 2 (110) oxides, we have performed ab-initio density functional theory (DFT) calculations [22] . We investigate TiO(001) rocksalt films of various thicknesses stacked pseudomorphically on top of a rutile TiO 2 slab oriented along the (110) direction. Several atomic configurations with different relative atomic positions between the titanium and oxygen atoms at both sides of the interface are considered ( Supplementary Notes and Supplementary Fig. 5 ). 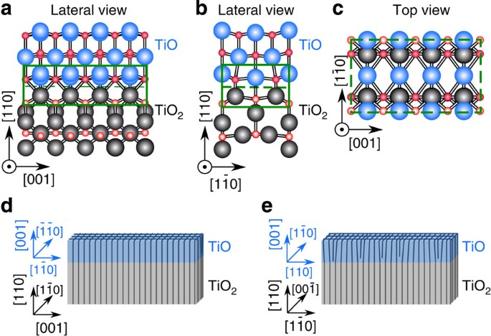Figure 4: Most stable surface configuration calculated with DFT. (a,b) Side views along the [10] and [001] directions, respectively, referred to the TiO2crystal lattice. The interfacial region separating both oxides is marked with a green rectangle. Ti and O atoms are depicted in small red (pink) and big blue (grey) balls, respectively, in the TiO (TiO2) crystal. (c) Top view of the interface, where just the upmost layer of the TiO2substrate and the first layer of the TiO thin film are visualized. (d,e) Schemes of the atomic planes at the interface between the TiO2(110) substrate and the TiO(001) layer along two perpendicular directions. Tilted regions of the TiO layer are present mainly because of the poor matching between both lattices along the [10] direction. Figure 4a–c shows the structure of the lowest energy configuration, which is favoured by 350 meV per interface TiO unit over the second lowest energy configuration. It presents a good chemical and structural matching and, despite distortions, the interfacial Ti cations are either six- or fivefold coordinated, close to the Ti coordination in both oxides, while the oxygen atoms are fivefold coordinated. The [10] uniaxial tensile strain endured by the pseudomorphic TiO(001) layer induces a buckling at the interface, which is released in five or six layers within the TiO. Besides, and in agreement with the experimental observation, the out-of-plane TiO distance slightly increases with the interface distance ( Supplementary Fig. 6 ). This contraction of the TiO bonds at the interface is due to the charge transfer from the TiO towards the TiO 2 , resulting in a metallic interface ( Supplementary Fig. 7 ). The lowest energy configuration shown in Fig. 4 has a work of separation of γ int =3.2 J m −2 , corresponding to a rather stable interface. This stability can be attributed to the good structural matching of the two lattices [23] and favours the formation of a rocksalt TiO film in registry with the substrate. Figure 4: Most stable surface configuration calculated with DFT. ( a , b ) Side views along the [10] and [001] directions, respectively, referred to the TiO 2 crystal lattice. The interfacial region separating both oxides is marked with a green rectangle. Ti and O atoms are depicted in small red (pink) and big blue (grey) balls, respectively, in the TiO (TiO 2 ) crystal. ( c ) Top view of the interface, where just the upmost layer of the TiO 2 substrate and the first layer of the TiO thin film are visualized. ( d , e ) Schemes of the atomic planes at the interface between the TiO 2 (110) substrate and the TiO(001) layer along two perpendicular directions. Tilted regions of the TiO layer are present mainly because of the poor matching between both lattices along the [10] direction. Full size image The above results suggest that, at the very initial stages of ion bombardment, the preferential sputtering of oxygen atoms renders a chemically reduced rutile crystalline structure, which transforms into a disordered phase for intermediate doses. For a sufficiently high concentration of oxygen vacancies, the rutile structure is no longer stable and a single-crystalline rocksalt TiO phase emerges according to the new stoichiometry, with a moderate concentration of Ti 3+ and Ti 4+ cations. This transformation is favoured by the good matching at the interface along the [001] direction of TiO 2 . However, the lattice match is not perfect along the [10] direction, where the misfit is about 10%. Misfit accommodation in oxides is complex and can comprise several mechanisms [24] . A most plausible model involving dislocations is compatible with our experimental observations. The existence of dislocations along the [10] direction of TiO 2 and, therefore, the presence of extra {110} half-planes in the rocksalt structure (which is indeed its slip direction [25] ) would induce a relaxation and bending of the adjacent planes which, for the case of a thin film, justifies the asymmetry of the rocking curves and the elongation of the LEED spots. Regarding the thickness of the TiO layer, it is larger than the average depth where most of the vacancies are created, which is calculated to be R P =3.8±2.0 nm ( Supplementary Fig. 3 ) [26] . But, considering replacement sequences, interstitials can be created deeper than R P (ref. 17 ) and, furthermore, diffusion mechanisms can be also invoked. It must be also remarked that the energetic ion beam locally increases the temperature of the surface of the sample and assists diffusion processes. Mass transport in reduced TiO 2 surfaces is mainly related to the mobility of Ti cations [27] , [28] , which in the form of interstitials are present in the bulk and mostly in the bombarded layer. While it is difficult to devise the kinetics of the formation process of the thin film, a conceivable model could consider the migration of these interstitials to the TiO(001)/TiO 2 (110) interface (driven by a strong chemical gradient). At the interface they would incorporate to the dioxide and locally transform it into monoxide. The result would be the advancement of the interface towards the TiO 2 bulk. In any case, the thickness of the modified layer must eventually saturate once the diffusion length of the species is not sufficiently long to compensate for the receding surface (material is being continuously removed by the ion beam). Then a steady state is reached, as we have indeed observed experimentally. Notwithstanding the details of the kinetics, the transformation of the pristine rutile dioxide into the rocksalt monoxide is thermodynamically ruled by the stability of the interface and probably assisted by the increased local temperature. We show here that, in contrast to previous works, the surface of ion-bombarded oxides cannot always be simply described as a reduced and defective oxide region, but rather as a thin film of a new oxide. In particular, the results presented here demonstrate that ion bombardment induces the formation of a single-crystalline rocksalt TiO(001) thin film in registry with the rutile TiO 2 (110) substrate underneath. Our work clarifies the role of ion bombardment on the atomic structure and establishes a new route to generate, for certain cases, heterostructures and interfaces between an oxide and its corresponding suboxide, in a relatively simple and controlled way. LEIB shows in this case a new technologically relevant capability, applied in particular to the formation of a TiO(001)/TiO 2 (110) interface, whose functional properties well deserve to be further explored. Experimental methods Rutile TiO 2 (110) single crystals, from Surface Preparation Laboratories, were ion-bombarded in a UHV chamber, where they were also characterized with LEED and Auger spectroscopy. The Ar + flux was 4.2 × 10 16 ions·h −1 ·cm −2 and the total dose was 8.4 × 10 16 ions·cm −2 . Grazing-incidence XRD was carried out at the six-circle diffractometer installed at the BM25-SpLine beamline (Branch B) at the European Radiation Facility (ESRF). Diffraction measurements were performed using the constant grazing incidence geometry with a fixed energy of 14 keV. STEM data were acquired in an aberration-corrected JEOL JEM-ARM200cF electron microscope equipped with a cold field emission gun and a Gatan Quantum spectrometer. Computational methods DFT calculations were performed using the projector augmented plane wave method within the PBE approximation for the exchange-correlation functional, as implemented in the Vienna ab-initio Simulation Package (VASP) [22] , [29] , [30] . The TiO(001)/TiO 2 (110) interface was modelled using a periodic slab geometry containing a vacuum region of around 12 Å to inhibit the interaction between neighbouring surfaces. The TiO/TiO 2 slabs contained seven layers (ML) of TiO 2 and the number of TiO layers ranged from 1 to 17 ML, each layer including two unit cells. The 3 p semicore states of Ti were included in the valence states. In all the calculations the in-plane lattice parameters were fixed to the experimental 2.95 and 6.49 Å of bulk rutile TiO 2 (ref. 31 ), while the perpendicular lattice constant was optimized. A kinetic energy cutoff of 400 eV was used, and the interface Brillouin zone was sampled employing a 11 × 5 × 1 k -point grid. All the atomic positions are fully relaxed until atomic forces are <0.01 eV Å −1 . We have calculated the TiO and TiO 2 bulk oxides, obtaining satisfactory electronic and structural properties compared with previous works [32] , [33] . How to cite this article: Pabón, B. M. et al . Formation of titanium monoxide (001) single-crystalline thin film induced by ion bombardment of titanium dioxide (110). Nat. Commun. 6:6147 doi: 10.1038/ncomms7147 (2015).